High specificity in plant leaf metabolic responses to arbuscular mycorrhiza The chemical composition of plants (phytometabolome) is dynamic and modified by environmental factors. Understanding its modulation allows to improve crop quality and decode mechanisms underlying plant–pest interactions. Many studies that investigate metabolic responses to the environment focus on single model species and/or few target metabolites. However, comparative studies using environmental metabolomics are needed to evaluate commonalities of chemical responses to certain challenges. We assessed the specificity of foliar metabolic responses of five plant species to the widespread, ancient symbiosis with a generalist arbuscular mycorrhizal fungus. Here we show that plant species share a large ‘core metabolome’ but nevertheless the phytometabolomes are modulated highly species/taxon-specifically. Such a low conservation of responses across species highlights the importance to consider plant metabolic prerequisites and the long time of specific plant-fungus coevolution. Thus, the transferability of findings regarding phytometabolome modulation by an identical AM symbiont is severely limited even between closely related species. Plants are not at all static or easily predictable systems, but are highly dynamic in their chemical composition, which is modulated by environmental factors [1] , [2] . The phytometabolome is a snapshot of the complete set of metabolites of a plant, representing the metabolic phenotype [2] , [3] . The specific metabolic composition determines the quality of herbs used as food, medicine or industrial materials. Moreover, being downstream of the transcriptome and proteome, the metabolome is closest to diverse biological functions and thus decisive for ecological interactions between plants, their enemies and beneficial organisms. A thorough understanding of phytometabolome modulation is necessary to eventually decode mechanisms underlying changes in plant quality evoked by an identical challenge. Traditionally, targeted analyses focused on the analysis of a few well-characterized metabolites to determine plant responses, thereby missing much of the complete (chemical) picture [4] . However, in the postgenomic era of systems biology, metabolomic approaches are increasingly used to assess the metabolomes of organisms in a comprehensive, unbiased way [1] , [2] , sometimes revealing unexpected regulation patterns [3] . By combining several analytical platforms, assessments of metabolic phenotypes including metabolites from various chemical classes are now feasible [3] . However, most knowledge on modulation considering a substantial set of metabolites relies on studies of few model plant species (for example, Arabidopsis thaliana [5] , Lotus spec. [6] , [7] , Medicago truncatula [8] , Plantago spec. [4] , [9] , [10] ) and the transferability of findings from these models to other plant systems is debatable. Since plant species [7] , [11] , [12] , [13] and even conspecifics [14] differ in their metabolomes, metabolic prerequisites of species have to be taken into account to delineate common from species-specific changes in response to an identical challenge. Arbuscular mycorrhiza (AM) the mutualistic interaction between plants and root colonizing arbuscular mycorrhizal fungi (AMF)—offers a suitable system to investigate the specificity of phytometabolome responses to an identical challenge for the following reasons. First, AMF should modulate the plant metabolome by improving water uptake and nutrition of the host plant mainly due to elevated phosphate supply, by acting as additional sink for plant-derived photosynthates (up to 20% of plant-fixed carbon) and by influencing photosynthesis, thus being tightly connected to the host’s physiology [15] . Second, mycorrhizal associations are ancient and phylogenetically widespread (in >80% of land plant species) [15] , thereby being of major importance for most plants in different natural and agricultural ecosystems. Third, arbuscular mycorrhizas are of considerable agricultural importance, as AMF enhance nutritional values and yields of crops, modulate plant pest and stress resistance, and influence global C and P cycling, ecosystem services, and primary productivity [15] , [16] , [17] . In contrast to the roots, whose metabolism under AM symbiosis is well characterized [8] , systemic effects of AMF, whose morphological structures are restricted to the roots, on shoot metabolic phenotypes are sparse and were mainly studied for certain targets or metabolomes of single species yet [6] , [18] , [19] , [20] , [21] , [22] , [23] . To determine the extent of common versus species-specific modulation patterns of foliar metabolomes by a widespread generalist AMF, we performed a comparative multi-species environmental metabolomic [1] approach including five model and non-model plant species with different phylogenetic relatedness. Although the five plant species share between 18 and 45% of their polar metabolome, only few common metabolic modulations occur. We show that the high degree of species-specificity in response to the identical AMF impedes the transferability of findings even between closely related species. Comparable mycorrhizal establishment We included five mycotrophic plant species in our comparative multi-species metabolomic approach to evaluate the commonality versus specificity of systemic responses to the AMF species Rhizophagus irregularis , which is closely related to some world-wide [24] distributed AMF species. Mycorrhizal plants (AM) were compared with control plants (NM), which received a sterilized inoculum and a microorganism filtrate ( n =10 plants per treatment and plant species). Plantago lanceolata ( Pl ) and P. major ( Pm , Plantaginaceae) were chosen for within-genus comparisons and as they are model species in ecological studies with their metabolomes being well-characterized [4] , [9] , [10] . Veronica chamaedrys ( Vc , Plantaginaceae) was included to allow between-genus comparisons within the same plant family. Medicago truncatula ( Mt , Fabaceae), for which the association with root symbionts is well characterized [8] , [25] , represented another dicot family, whereas Poa annua ( Pa , Poaceae) was included as representative of the monocots. The chosen species are herbaceous with comparable statures and share largely similar habitats. We ensured that both the internal root colonization and the extra-radical hyphal extension developed similarly in all plant species with comparable slopes reaching a stable plateau of ~80% internal fungal colonization (in P. annua ~60%) at 62 days post inoculation (d.p.i.) ( Fig. 1a–d , Supplementary Data 1 ). Hyphal networks, arbuscules (sites for the exchange of nutrients and photosynthates) and vesicles (fungal storage organs) were comparably well established in the roots of all plant species, indicating functional nutritional plant–fungus interfaces ( Fig. 1e , Supplementary Data 1 ). Moreover, at 62 d.p.i., aboveground biomass slightly differed between species but not between NM and AM plants within each species ( Fig. 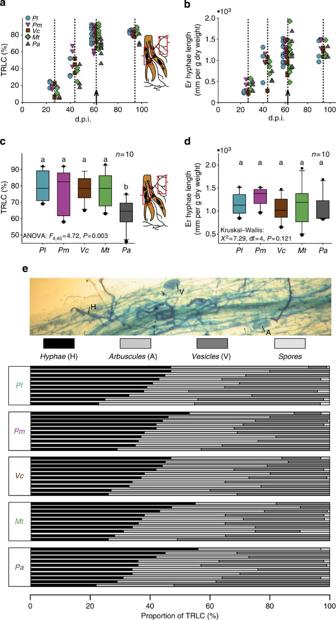Figure 1: Comparable mycorrhizal symbiosis in all tested plant species at 62 days post inoculation. (a) Development of total root length colonization (TRLC) of mycorrhizal plants over time (d.p.i., days post inoculation). (b) Length of extra-radical (er) hyphae of mycorrhizal plants over time. (c) TRLC of mycorrhizal plants at 62 d.p.i. as Box-Whisker plots. Different letters indicate significant differences inpost-hocTukey HSD tests (P<0.05). (d) Length of er hyphae of mycorrhizal plants related to the dry weight of the growth substrate at 62 d.p.i. as Box-Whisker plots. Different letters indicate significant differences inpost-hocKruskal mc tests (P<0.05). (e) Proportions of fungal structures for individual replicates of mycorrhizal plants at 62 d.p.i. (a–e)Pl,Plantago lanceolata;Pm,Plantago major;Vc,Veronica chamaedrys;Mt,Medicago truncatula;Pa,Poa annua. The Box-Whisker plots show the median (horizontal line), the interquartile range (box) and the whiskers (extending to the 5 and 95% percentile, respectively);n=10 biological replicates at 62 d.p.i. 2 , Table 1 ). This means that under the fertilization regime applied soil nutrients were limited enough to allow mycorrhizal establishment in inoculated plants, but did not lead to severe nutrient limitation of control plants. Concordantly, the proportion of flowering plants was similar or equal between NM and AM plants within each species ( Pl : 40% for both; Pm : 100% for both; Vc : 0% for both; Mt : 100% for both; Pa : 50% for NM and 40% for AM plants). Both the similar AMF establishment between species and the lack of mycorrhizal growth responses within species allowed us to compare the metabolic phenotypes of the different plants at 62 d.p.i. in a valid way, excluding the confounding effects of differences in developmental stages of the leaves or plant reproductive status. Figure 1: Comparable mycorrhizal symbiosis in all tested plant species at 62 days post inoculation. ( a ) Development of total root length colonization (TRLC) of mycorrhizal plants over time (d.p.i., days post inoculation). ( b ) Length of extra-radical (er) hyphae of mycorrhizal plants over time. ( c ) TRLC of mycorrhizal plants at 62 d.p.i. as Box-Whisker plots. Different letters indicate significant differences in post-hoc Tukey HSD tests ( P <0.05). ( d ) Length of er hyphae of mycorrhizal plants related to the dry weight of the growth substrate at 62 d.p.i. as Box-Whisker plots. Different letters indicate significant differences in post-hoc Kruskal mc tests ( P <0.05). ( e ) Proportions of fungal structures for individual replicates of mycorrhizal plants at 62 d.p.i. ( a – e ) Pl , Plantago lanceolata ; Pm , Plantago major ; Vc , Veronica chamaedrys ; Mt , Medicago truncatula ; Pa , Poa annua . The Box-Whisker plots show the median (horizontal line), the interquartile range (box) and the whiskers (extending to the 5 and 95% percentile, respectively); n =10 biological replicates at 62 d.p.i. 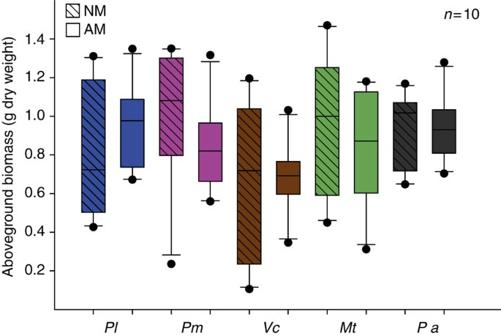Figure 2: Lack of mycorrhizal growth responses. Total aboveground biomass of control (NM) and mycorrhizal (AM) plants as Box-Whisker plots showing the median (horizontal line), the interquartile range (box) and the whiskers (extending to the 5 and 95% percentile, respectively) at 62 d.p.i. (days post inoculation).Pl,Plantago lanceolata;Pm,Plantago major;Vc,Veronica chamaedrys;Mt,Medicago truncatula;Pa,Poa annua;n=10 biological replicates. Full size image Figure 2: Lack of mycorrhizal growth responses. Total aboveground biomass of control (NM) and mycorrhizal (AM) plants as Box-Whisker plots showing the median (horizontal line), the interquartile range (box) and the whiskers (extending to the 5 and 95% percentile, respectively) at 62 d.p.i. (days post inoculation). Pl , Plantago lanceolata ; Pm , Plantago major ; Vc , Veronica chamaedrys ; Mt , Medicago truncatula ; Pa , Poa annua ; n =10 biological replicates. Full size image Table 1 Results of generalized linear model fitting plant biomass at 62 days post inoculation. Full size table Metabolic phenotypes of plant species The total leaf phosphorus content did not significantly differ between plant species ( Fig. 3a ; Supplementary Data 1 ), as indicated by deletion of the factor ‘ Species ’ during Akaike’s information criterion-driven model simplification of a generalized linear model ( Table 2 ). In contrast, carbon and nitrogen content differed significantly between species, with V. chamaedrys showing the highest values for both elements ( Fig. 3b , Table 2 , Supplementary Data 1 ). In addition, N was influenced by the total aboveground biomass of the plants ( Table 2 ). 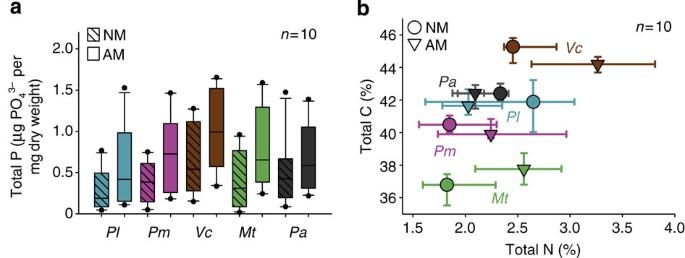Figure 3: Arbuscular mycorrhiza increases foliar P but not C and N in all tested species. (a) Total P (PO43−of mineralized leaves) of control (NM) and mycorrhizal (AM) plants ofPl(Plantago lanceolata),Pm(Plantago major),Vc(Veronica chamaedrys),Mt(Medicago truncatula) andPa(Poa annua) as Box-Whisker plots showing the median (horizontal line), the interquartile range (box) and the whiskers (extending to the 5 and 95% percentile, respectively). (b) C and N contents of leaves, given as median with 25 and 75% percentiles. (a,b)n=10 biological replicates. A comprehensive metabolomic approach combining targeted metabolite profiling of carbohydrates, organic acids, sugar alcohols (via gas chromatography coupled to mass spectrometry, GC–MS) and amino acids (via high-performance liquid chromatography coupled to fluorescence detection, HPLC-FL), and untargeted metabolic fingerprinting (via ultra-HPLC coupled with time of flight MS, uHPLC-ToF-MS) of methanolic leaf extracts revealed in total 6,870 metabolic features (57 per GC–MS, 22 per HPLC-FL, 6,791 per uHPLC-ToF-MS) including metabolites, analytes and mass traces (encoded by chromatographic retention time and specific mass, Table 3 ). Thereof, we could identify various primary and secondary metabolites from different chemical classes broadly covering the main plant metabolic pathways ( Table 3 ). However, the number of detected features per sample differed significantly between species, with V. chamaedrys having the highest and P. annua the lowest numbers ( Fig. 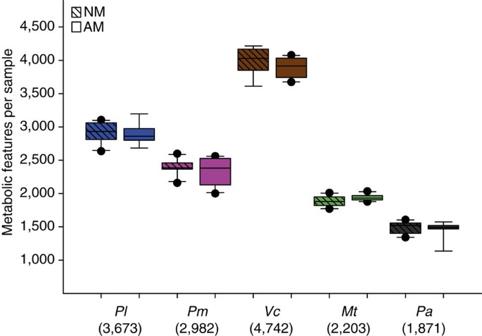Figure 4: Numbers of metabolic features detected in leaf samples. Across all species, 6,870 metabolic features were found. Numbers of metabolic features in control (NM) and mycorrhizal (AM) plants ofPl(Plantago lanceolata),Pm(Plantago major),Vc(Veronica chamaedrys),Mt(Medicago truncatula) andPa(Poa annua) as Box-Whisker plots showing the median (horizontal line), the interquartile range (box) and the whiskers (extending to the 5 and 95% percentile, respectively). For each species, the total number of features found is given in brackets;n=9 to 10 biological replicates. 4 , Table 4 , Supplementary Data 1 ). Including various carbohydrates, organic acids, amino acids and others, 850 metabolic features were shared between all plant species (occurring mostly in both NM and AM plants, with few exceptions detected in one treatment group only, see below) thus representing an overlapping ‘core metabolome’ ( Fig. 5a ), accounting for high proportions of the polar metabolomes of individual plant species (23% for P. lanceolata , 29% for P. major , 18% for V. chamaedrys , 39% for Medicago truncatula , 45% for P. annua ). Beyond that, metabolic phenotypes comprised many features being specific for single species like, for example, the sugar alcohol mannitol, which was only detectable in V. chamaedrys , and the cyclic polyols pinitol and ononitol being characteristic for M. truncatula ( Fig. 5a ). Other features mirrored phylogenetic relationships, such as the sugar alcohol sorbitol, which was common for the genus Plantago , and aucubin and verbascoside, which were found exclusively in the Plantaginaceae ( Fig. 5a ). Many further metabolic features may be determined using additional platforms. Figure 3: Arbuscular mycorrhiza increases foliar P but not C and N in all tested species. ( a ) Total P (PO 4 3− of mineralized leaves) of control (NM) and mycorrhizal (AM) plants of Pl ( Plantago lanceolata ), Pm ( Plantago major ), Vc ( Veronica chamaedrys ), Mt ( Medicago truncatula ) and Pa ( Poa annua ) as Box-Whisker plots showing the median (horizontal line), the interquartile range (box) and the whiskers (extending to the 5 and 95% percentile, respectively). ( b ) C and N contents of leaves, given as median with 25 and 75% percentiles. ( a , b ) n =10 biological replicates. Full size image Table 2 Results of generalized linear models fitting foliar elemental contents of five plant species with and without mycorrhiza. Full size table Table 3 List of identified metabolites. * Full size table Figure 4: Numbers of metabolic features detected in leaf samples. Across all species, 6,870 metabolic features were found. Numbers of metabolic features in control (NM) and mycorrhizal (AM) plants of Pl ( Plantago lanceolata ), Pm ( Plantago major ), Vc ( Veronica chamaedrys ), Mt ( Medicago truncatula ) and Pa ( Poa annua ) as Box-Whisker plots showing the median (horizontal line), the interquartile range (box) and the whiskers (extending to the 5 and 95% percentile, respectively). For each species, the total number of features found is given in brackets; n =9 to 10 biological replicates. Full size image Table 4 Results of generalized linear model fitting the number of metabolic features detected in leaf samples. 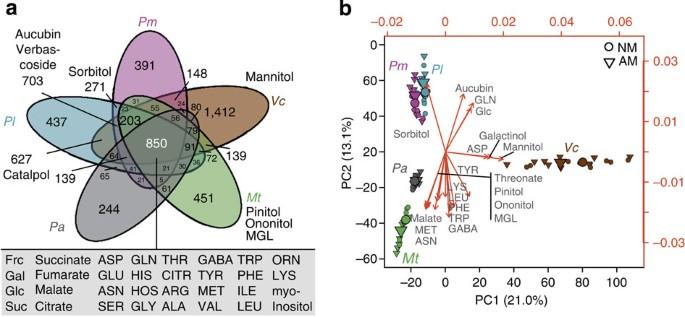Figure 5: Plant species differ in their foliar metabolomes. (a) Numbers of metabolic features occurring and overlapping inPl(Plantago lanceolata),Pm(Plantago major),Vc(Veronica chamaedrys),Mt(Medicago truncatula) andPa(Poa annua) as Venn diagram. Cardinalities are encoded by font size, some identified features are labelled (abbreviations:Table 3). (b) Metabolic pattern of control (NM) and mycorrhizal (AM) plants as principal component analysis (PCA) with scores (black axis, symbols), the 20 highest loadings (red axis, arrows) of identified features, the percent total variance explained by the PCs in brackets, and the median scores as larger symbols for each group; (a,b)n=9 to 10 biological replicates. Full size table Figure 5: Plant species differ in their foliar metabolomes. ( a ) Numbers of metabolic features occurring and overlapping in Pl ( Plantago lanceolata ), Pm ( Plantago major ), Vc ( Veronica chamaedrys ), Mt ( Medicago truncatula ) and Pa ( Poa annua ) as Venn diagram. Cardinalities are encoded by font size, some identified features are labelled (abbreviations: Table 3 ). ( b ) Metabolic pattern of control (NM) and mycorrhizal (AM) plants as principal component analysis (PCA) with scores (black axis, symbols), the 20 highest loadings (red axis, arrows) of identified features, the percent total variance explained by the PCs in brackets, and the median scores as larger symbols for each group; ( a , b ) n =9 to 10 biological replicates. Full size image In addition to these qualitative differences, we included quantitative data as meaningful information in our analyses. A pronounced distinction of metabolic phenotypes between species was depicted by principal component analysis (PCA; Fig. 5b ), again revealing highest metabolic similarities between both Plantago species. Apart from the species-specific metabolites, quantitative differences in compounds separated the phytometabolomes, with, for example, many amino acids being higher concentrated in the grass P. annua compared with the Plantago species (loadings in Fig. 5b ). In conclusion, the plant species shared a large proportion of metabolic features but exhibited also distinct metabolic profiles characterized by both qualitative and quantitative differences, partly reflecting phylogenetic relationships. Whereas in the core metabolome shared by all plant species common, that is, species-independent, plant responses to an identical challenge could potentially be found, features only occurring in one or few species may contribute to species- or taxon-specific changes. Species-specific AM effects on plants Total foliar phosphorus content was significantly increased in AM compared with NM plants in all plant species ( Fig. 3a , Table 2 ), thus representing a common phytometabolome response to AMF root colonization. This finding confirms that the symbiotic associations were not only morphologically well established ( Fig. 1 ) but also functional. In contrast to phosphorus, AM-mediated effects on leaf carbon and nitrogen were less pronounced and differed between species ( Fig. 3b ), as indicated by significant Species × Treatment interaction terms in the minimal adequate generalized linear models (GLMs) ( Table 2 ). Remarkably, although phosphorus increased significantly in all species, effects of AMF root colonization were only marginally visible in the leaf metabolic phenotypes ( Fig. 5b ) indicating that the large chemical differences between species superimposed within-species AMF effects. Thus, we further traced AM effects by within-species analyses of metabolome modulation patterns. Therefore, a metabolic feature was regarded as modulated by AM if its concentration significantly differed between NM and AM plants (Mann–Whitney U -test, P <0.05) and if additionally a fold change of <0.67 (decrease in metabolite pool size) or >1.5 (increase in metabolite pool size) in intensity in AM compared with NM plants were detected ( Fig. 6a ). According to these thresholds, considerable fractions of the leaf metabolomes were modulated by AMF colonization of the roots (coloured symbols in Fig. 6a ), covering different parts of the plant metabolic pathway network. However, overall responsiveness to mycorrhization markedly differed between plant species. Medicago truncatula was most responsive to AM with 14.7% of its metabolic features being modulated, whereas the Plantaginaceae species exhibited an intermediate responsiveness ( P. lanceolata : 5.8%, P. major : 5.4%, V. chamaedrys : 5.7%) and the grass was least responsive (1.7%) to AM symbiosis. Only very few (<1% of features within each plant species) were changed in a qualitative manner by AM, that is, exclusively found in either NM or AM plants. Moreover, species differed in their metabolome modulation patterns, that is, the proportions of features being decreased versus increased ( Fig. 6a,b ). Remarkably, a comparison of the modulation of individual metabolic features between species revealed that most metabolic responses to AM were highly species-specific ( Fig. 6b ). Features modulated by AM in one species were either not detectable in other species (grey cells, Fig. 6b ) or present, but were changed in the opposite direction or not modulated at all. For example, the pool size of the secondary metabolite catalpol was highly increased by AM in P. lanceolata , whereas it was slightly decreased in V. chamaedrys ( Fig. 6b , feature cluster b 3 , Fig. 6c ). Nevertheless, at least some common responses of metabolites to AMF colonization could be found within the dicotyledonous species (for example, feature clusters b 1 , b 2 in Fig. 6b ). Most notably, several organic acids from the citric acid cycle (citrate, malate, fumarate; partly: succinate, isocitrate) decreased in pool sizes under AM conditions in P. lanceolata , P. major , V. chamaedrys and M. truncatula , but increased in the grass P. annua ( Fig. 6b,c ). Moreover, some amino acids were significantly increased under AM conditions in certain plant species, but with fold changes below the defined threshold ( Fig. 6c ). Thus, analyses of metabolic modulation patterns revealed that species-specific metabolic shifts on AMF colonization outbalance common, species-independent responses by far, with the latter ones being nevertheless found but mainly restricted to the dicotyledonous species. 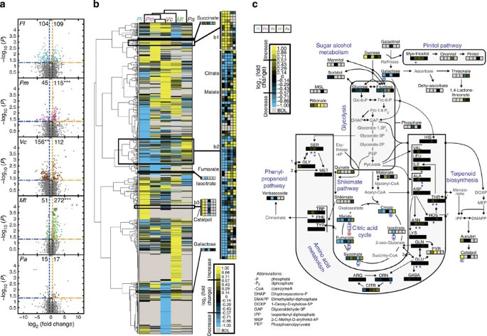Figure 6: Phytometabolomes are modulated by mycorrhization species-specifically. (a) Modulated features as coloured symbols outside the cutoff-lines in volcano plots (Mann–WhitneyU-test: unadjustedP<0.05; fold change <0.67 for decrease in metabolite pool size, left; >1.5 for increase in metabolite pool size, right). Crosses indicate significance after adjustment of thePvalues (FDR=0.05) of the Mann–WhitneyU-tests. The feature numbers of de-versusincreased features were compared (χ2-tests; **P<0.01, ***P<0.001). (b) Average linkage hierarchical cluster heatmap (Pearson correlation) of 975 features modulated in minimum one species. BDL, below detection limit. (c) The plant metabolic pathway map displaying mycorrhiza-mediated changes of different metabolites. Not all reactions and reaction products are shown (dashed arrows, intermediates omitted), the full names are given on left-hand side and inTable 3, the heatmap strips (fold changes) are colour coded. Asterisks indicate significance (Mann–WhitneyU-tests; *P<0.05, **P<0.01, ***P<0.001; blue, according to unadjustedP; red, adjustedP), borders around the asterisks indicate fold changes <0.67 or >1.5. (a–c)Pl,Plantago lanceolata;Pm,Plantago major;Vc,Veronica chamaedrys;Mt,Medicago truncatula;Pa,Poa annua. Means ofn=9 to 10 biological replicates. Figure 6: Phytometabolomes are modulated by mycorrhization species-specifically. ( a ) Modulated features as coloured symbols outside the cutoff-lines in volcano plots (Mann–Whitney U -test: unadjusted P <0.05; fold change <0.67 for decrease in metabolite pool size, left; >1.5 for increase in metabolite pool size, right). Crosses indicate significance after adjustment of the P values (FDR=0.05) of the Mann–Whitney U -tests. The feature numbers of de- versus increased features were compared ( χ 2 -tests; ** P <0.01, *** P <0.001). ( b ) Average linkage hierarchical cluster heatmap (Pearson correlation) of 975 features modulated in minimum one species. BDL, below detection limit. ( c ) The plant metabolic pathway map displaying mycorrhiza-mediated changes of different metabolites. Not all reactions and reaction products are shown (dashed arrows, intermediates omitted), the full names are given on left-hand side and in Table 3 , the heatmap strips (fold changes) are colour coded. Asterisks indicate significance (Mann–Whitney U -tests; * P <0.05, ** P <0.01, *** P <0.001; blue, according to unadjusted P ; red, adjusted P ), borders around the asterisks indicate fold changes <0.67 or >1.5. ( a – c ) Pl , Plantago lanceolata ; Pm , Plantago major ; Vc , Veronica chamaedrys ; Mt , Medicago truncatula ; Pa , Poa annua . Means of n =9 to 10 biological replicates. Full size image The current study points out that systemic phytometabolome responses to root colonization by the same AMF species with similar extent of symbiotic establishment are highly plant species-specific with only low degrees of conservation across species. Moreover, metabolome responses only marginally reflected phylogeny within the dicotyledonous species, but some general differences between dicots and the monocot emerged. Importantly, we could ensure that the metabolic responses to AMF root colonization are not confounded by differences in leaf developmental stages and plant reproductive status, as under the conditions applied no mycorrhizal growth responses in AM compared with NM plants occurred. Nevertheless, the species-independent common increase in foliar phosphorus content clearly indicates a response to AM, which is consistent with other studies [26] , [27] . However, the AM-mediated improved phosphate uptake [15] did not translate to common metabolome responses across the investigated species. This result is particular striking, as the high proportion of metabolic features shared between some or all species (‘core metabolome’) would potentially allow for many overlapping responses. However, in line with our findings, AM effects on leaf essential oil composition of mint and oregano were found to be plant species-specific as well [26] . Also, species-specific metabolome responses to abiotic factors were described (for example, response of Lotus [7] and Eucalyptus [28] species to water availability), which may, however, be confounded by different tolerance of the species to the abiotic stressor under investigation or different plant size. The high species-specificity of responses to AM may be interpreted in the context that the AM symbiosis dates back to the earliest land plants [15] . This ancient origin of the symbiotic fungi allowed individual plant species to coevolve with the AMF from the corresponding plant speciation event on and to develop plant species-specific adaptations mirrored in specific metabolome changes under symbiosis, with this specificity being maintained, although the AMF associated with other plant species in parallel. In accordance, plant growth responses to AMF were described to be relatively open to evolutionary change with limited phylogenetic constraints [29] . Thus, metabolic modulation by AMF in one plant species only allows limited predictions for responses to the same fungal symbiont in another species. Those metabolic features present exclusively in one or a subset of the plant species contributed to specific responses, highlighting the need to take metabolic backgrounds of plant species into account in comparative environmental phytometabolome studies. Indeed, plant species have distinct metabolic phenotypes due to qualitative and quantitative differences in metabolites [7] , [11] , [12] , [13] emerging from different evolutionary selection pressures and ecological niches occupied by the respective species. The high responsiveness of the Fabaceae M. truncatula may be attributed to its extraordinary high affinity to root symbionts, including AMF but also nodule-forming rhizobia [25] (not detected under our experimental conditions), somehow priming the plants to strongly respond to these endosymbionts. In contrast to the high proportion of species-specific changes, the decrease in organic acids of the citric acid cycle in AM plants was a common response in all dicots of our study. This finding may be explained by a negative impact of AM symbiosis on central catabolism and was also detected in leaves of Lotus japonicus [6] . However, in L. japonicus , moreover, a decrease in amino acids was found, which may be specific to this species. The changes in catabolic processes may be related to the carbon sink strength imposed by the AMF. The contrary response of the grass, P. annua , regarding organic acids corresponds well with increases of organic acids of the citric acid cycle found in maize [30] and barley [31] (Poaceae) leaves under mycorrhizal conditions and may point to general differences in metabolism of dicots versus monocots. In addition, the lower fungal root colonization in the grass compared with the dicot species ( Fig. 1 ), which is consistent with other studies [29] , may have contributed to the distinct response patterns observed. The differences in colonization levels may reflect contrasting strategies of nutrient acquisition [32] with the grass species allocating more in an extensive root system and the dicots investing more in symbiotic structures. The implications of our study may be relevant for future studies on plant chemistry and the ecological interactions in which plants are involved. First of all, it is advisable to supplement the analysis of only few target metabolites with multi-platform metabolomic approaches to gain an unbiased, comprehensive view of plant metabolome modulation. Second, to characterize plant responses to an identical challenge, various species preferably of different plant families should be included in comparative approaches to account for different metabolic backgrounds and uncover common versus species-specific responses. Indeed, our results highlight that findings and conclusions obtained from one model species cannot be simply transferred to other model systems, even within congeners and not at all between di- and monocots, at least when considering this symbiotic interaction. More commonalities may occur in plant responses to abiotic stresses. In any case, care should be taken when transfer of scientific knowledge from non-crop model plant species to (closely related) crop species is pursued to improve plant chemistry. Third, the species-specificity of response to AMF root colonization has important implications for further ecological interactions between plants and their enemies or other beneficial organisms, as the AM-induced chemical changes probably affect the attractiveness and suitability of the plant host for other organisms. For example, the AM-induced increase of foliar catalpol, a secondary metabolite involved in direct plant defence [33] , which was concordantly reported in another study [34] , probably enhances plant resistance to generalist herbivores in P. lanceolata . Moreover, the high species-specificity of plant metabolome responses to AMF colonization demonstrated here may be one source of the high variation found in plant-mediated mycorrhiza effects on herbivores [35] . Future studies should address how the metabolic responses to AM change along with the establishment of the symbiotic interaction and which proportion of the responses can be attributed to the AM-mediated improved phosphorus status of the leaves. Mycorrhizal treatment of plants and plant harvest Seeds ( Plantago lanceolata L., Pl , and Plantago major L., Pm , Plantaginaceae, Blauetikett Bornträger GmbH, Offstein, Germany; Veronica chamaedrys L., Vc , Plantaginaceae, field sampled in the Swabian Alb, Germany; Medicago truncatula Gaertn., Mt , Fabaceae, cv. Jemalong wildtype line A17 (ref. 36 ); Poa annua L., Pa , Poaceae, Appels Wilde Samen GmbH, Darmstadt, Germany) were surface-sterilized with 70% ethanol, 100% sulphuric acid ( M. truncatula only) and 2% sodium hypochloride, and swelled in distilled water for 2 h. Then, the seeds were sown in a sterilized 3:2 mixture of leached swelling clay (pH 9.6, 0.9 g l −1 salt content, FiboExClay, Lamstedt, Germany) and sand (0.1–0.5 mm particle size, Quarzwerke GmbH, Frechen, Germany) and stored at 4 °C in the dark for 3 days. Afterwards, they were transferred to a climate chamber (20 °C, 16:8 L:D, 60–70% r.h.; Osram Fluora lamps, L 36W/77, Osram, Munich, Germany), and, 41 days after sowing, seedlings were transferred to 2 l pots (average photosynthetically active radiation of 208 μmol m −2 s −1 at pot height). Half of the plants (AM plants; randomly assigned to this treatment) of each species were inoculated with the arbuscular mycorrhizal fungus Rhizophagus irregularis (Blaszk., Wubet, Renker & Buscot) C. Walker & A. Schüßler comb. nov. [37] (Glomales, Glomeromycota; sand inoculum, pH 7, Inoq GmbH, Schnega, Germany). This fungal species was chosen, since as a generalist fungus it associates with many plant species thus allowing its use in a plant species-comparison approach. For inoculation, 200 ml of the living inoculum was mixed to the substrate and seedlings placed inside. Control (NM) plants received 200 ml of sterilized inoculum and a microorganism filtrate, which was obtained from the inoculum before sterilization by washing and filtrating the supernatant through a 20 μm sieve (Retsch, Haan, Germany). AM plants received the same amount of water instead. Pots were positioned in a randomized block design. All plants were watered thrice weekly as needed with the same volume for each pot and fertilized twice a week with increasing volumes of a modified ½ strength Hoagland [38] solution. One l of the fertilizer solution contained 2.5 ml 1 M Ca(NO 3 ) 2 , 2.5 ml 1 M KNO 3 , 1 ml 1 M MgSO 4 , 1.5 ml 0.1 M KH 2 PO 4 (reduced to 0.3 ml after inoculation for both NM and AM plants to mimic low-P soils and thus pronounced needs for AM symbiosis), 5 ml 0.01 M Fe(III)-citrate and 1 ml micronutrients: 0.001 M H 3 BO 3 , 0.0002 M NiCl 2 , 0.001 M ZnSO 4 , 0.0002 M MnCl 2 , 0.0005 M CuSO 4 , 0.0002 M CoCl 2 , 0.0002 M Na 2 MoO 4 . Plants were harvested for chemical analyses at 62 d.p.i., as preliminary tests had revealed that mycorrhizal colonization had well established and stabilized at this time point in all species (to confirm this for the current experiment, 3 × n =3 additional replicates of mycorrhizal plants of each species were prepared and mycorrhizal colonization determined at 27, 44 and 94 d.p.i., respectively). The leaves of the youngest third of the plants were harvested in the afternoon hours. Leaves were cut, weighed, immediately frozen in liquid N 2 to quench the metabolism and stored at −80 °C. Plant material was lyophilized, milled and leaf powder distributed for several analyses. All chemical analyses (see below) were done in randomized order of the samples. After harvesting aboveground plant parts, roots were carefully separated from the substrate, representative subsamples of each plant bleached in 10% KOH (15 min, 95 °C), acidified in 1% HCl for 5 min and stained with a solution containing one part trypan blue (0.4%, Sigma-Aldrich, Steinheim, Germany) and 40 parts of 2:1:2 lactic acid:glycerine:H 2 O for 48 h at room temperature. Stained roots were conserved in 4:2:1 lactic acid:glycerine:H 2 O at 4 °C in the dark. Total root length colonization (TRLC) was determined with the grid-line intersect method [39] counting at least 200 intersects per sample. Hyphal structures, arbuscules, vesicles and spores were counted separately. Root systems of M. truncatula were macroscopically monitored for nodule formation, but no nodules were detected and thus molecular interference with root nodule symbioses could be excluded. Lengths of extra-radical (er) hyphae were determined according to a published protocol [40] with some modifications. The substrate was dried at 40 °C for 48 h. Then, homogenous subsamples were submerged in distilled H 2 O amended with sodium hexametaphosphate (35 g l −1 ), shaken for 30 s, incubated for 30 min, filtered through a 40 μm sieve (Retsch) and redissolved in H 2 O. The solution was shaken for 5 s and after 1 min a subsample of the supernatant taken from a defined height, filtered (filtration system, Merck Millipore, Darmstadt, Germany; filter: 0.45 μm, d=25 mm) and stained on the filter with trypan blue solution (see above) for 5 min. Extra-radical hyphae were quantified microscopically by counting intersections with ocular crosslines of at least 200 stops (and averaging over several subsamples) according to equation (1). For both treatment groups (AM and NM), n =10 plants per species were prepared (biological replicates), as this sample size was found to be appropriate to assess phytometabolome changes [10] . Three samples had to be omitted due to technical problems, thus decreasing the sample size of the groups Pl (AM), Vc (NM) and Pa (AM) to n =9 for metabolome analyses. Determination of foliar elemental contents For determination of leaf phosphorus (P) content, leaf powder was treated with 200 μl 65% HNO 3 for 24 h and then mineralized via wet ashing at 200 °C with 2 × 200 μl 65% HNO 3 followed by 200 μl 60% HClO 4 . Samples were dissolved in 800 μl millipore-H 2 O and quantified photometrically at 690 nm (colorimetric ortho-PO 4 3− test 1–78, Macherey-Nagel, Düren, Germany) by averaging over duplicate or triplicate measurements using a KH 2 PO 4 calibration curve. Carbon (C) and nitrogen (N) content of leaf powder were determined by combustion with a C/N analyser (Vario MICRO Cube, Elementar Analysensysteme, Hanau, Germany). Metabolite profiling Targeted metabolite profiling of carbohydrates, organic acids and sugar alcohols was performed via GC–MS according to Kutyniok & Müller [5] and Schweiger et al. [10] Leaf powder was extracted in 1:2.5:1 chloroform:methanol:water (chloroform HPLC grade, AppliChem, Darmstadt, Germany; methanol LC-MS grade, Fisher Scientific, Loughborough, UK) adding ribitol (99%, Sigma-Aldrich) as internal standard. Subsamples of the methanol/water phase were dried under N 2 and derivatized by sequential methoximation and silylation at 37 °C for 60 and 30 min, respectively. Samples were analysed with a Focus GC-DSQII (Thermo Electron, Rodano, Italy) equipped with a VF-5 ms column (30 m × 0.25 mm i.d., 10 m guard column, Varian, Palo Alto, CA, USA) in electron impact positive ionization mode at 70 eV and a helium flow of 1.2 ml min −1 . Injection was carried out at 225 °C in 1:10 split mode at a transfer line temperature of 250 °C. The oven was programmed at 80 °C for 3 min, followed by a ramp of 5 °C min −1 to 325 °C. Masses from 50 to 750 m/z were detected in full scan mode. In addition, reference metabolites (from Sigma-Aldrich, AppliChem, Merck (Darmstadt, Germany), Roth (Karlsruhe, Germany), Macherey-Nagel) and n-alkanes (C8-C40, Sigma-Aldrich) were measured and Kováts retention indices [41] (RIs) determined. Furthermore, samples without biological material were measured as blanks. Metabolites were identified by comparison of their RIs, mass spectra, and characteristic qualifier and quantifier masses to references, the Golm metabolome database [42] , [43] , as well as mass spectral and retention time index (MSRI) libraries [44] . Peaks with a signal-to-noise ratio of at least three, which were absent in the blanks, were quantified in terms of peak areas in relation to ribitol with the software Xcalibur (Version 1.4. SR1, Thermo Electron). Amino acids and derivatives were analysed via HPLC-FL according to Schweiger et al. [10] Therefore, leaf powder was extracted in 80% cool methanol (4 °C) adding taurine (Sigma-Aldrich) as internal standard on ice. Samples were precolumn-derivatized with o-phthaldialdehyde (OPA, Sigma-Aldrich) with a mixture of 1 ml OPA-thiol-solution (1% OPA (m/v), 90.5% methanol (v/v), 9.5% 0.5 M borate buffer (pH 8.5), 1% 2-mercaptoethanol), 4 ml borate buffer (0.5 M, pH 8.5) and 4 ml methanol for 1 min and analysed by HPLC (Knauer, Berlin, Germany) equipped with a AccQ-Taq column (150 × 4 mm, Waters, Eschborn, Germany). For separation, a gradient of acetate-methanol solutions (eluent A: 50 mM acetate at pH 7.1, 19% methanol; eluent B: 50 mM acetate at pH 7.1, 75% methanol) at a flow rate of 1 ml min −1 was used starting with 0% B for 20 min, followed by a ramp to 100% B within 30 min, and ending with 100% B for 5 min, followed by a column equilibration cycle. Amino acid derivates were identified by comparison with standards and quantified by using response factors compared with taurine. Metabolic fingerprinting Untargeted metabolic fingerprinting via ultra-HPLC coupled with time of flight MS (uHPLC-ToF-MS) was performed according to Schweiger et al. [10] Leaf powder was extracted threefold in 90% cool methanol (4 °C) adding hydrocortisone (>98%, Sigma-Aldrich) as internal standard (pH 7) on ice. Samples were analysed by uHPLC-ToF-MS (1290 Infinity uHPLC and 6210 ToF, Agilent Technologies, Santa Clara, CA, USA) equipped with a C18 column (Kinetex XB-C18, 150 × 2.1 mm, 1.7 μm, with guard column; Phenomenex, Torrance, CA, USA) at a flow of 0.6 ml min −1 and 45 °C column temperature. For separation, a gradient from water with 0.1% formic acid (p.a., eluent additive for LC-MS,~98%, Sigma-Aldrich, eluent A) to acetonitrile (LC-MS grade, Fisher Scientific) with 0.1% formic acid (eluent B) was used, increasing from 2 to 30% B within 20 min, from 30 to 75% B within 9 min, and ending with a cleaning and column equilibration step. Measurements were taken in negative electrospray ionization mode with 350 °C gas temperature, 12 ml min −1 drying gas flow, 55 psig nebulizer pressure, −140 V fragmentor voltage, 3,500 V capillary voltage and 60 V skimmer voltage. Data were stored in centroid mode from 100 to 1,700 m/z . Samples containing no biological material were measured as blanks in between test samples. Data were exported from MassHunter Qualitative Analysis (version B.03.01, Agilent Technologies) after deisotoping. The xcms package [45] , [46] of R (version 2.15.2; R Core Team (2012). R: A language and environment for statistical computing. R Foundation for Statistical Computing, Vienna, Austria. ISBN 3-900051-07-0, URL http://www.R-project.org/ ) was used for peak picking, grouping of associated peaks and retention time correction with xset (method=‘centWave’, p.p.m.=15, profmethod=‘bin’, peakwidth=c (5,20), sntresh=10, prefilter=c (3, 500), fitgauss=TRUE), retcor (method=‘obiwarp’), and group (bw=5, minfrac=0.5, mzwid=0.015) using only peaks eluting within the first 28 min. Peak intensities were related to hydrocortisone and only peaks with intensities >100 times the intensity in the blanks (averaged per median) considered. Metabolic features were identified by comparison of retention times and accurate masses to reference standards (aucubin, catalpol and verbascoside, Phytoplan, Heidelberg, Germany, >99%). Data processing and statistics Data from all analytical platforms were combined retaining only those features, which occurred in at least 50% of the replicates of one group after processing. Features that occurred in <20% of the samples of one species were omitted for this species. Peak intensities were related to the dry weight of the samples and transformed by log 10 (peak intensity +1). If not otherwise stated, statistical analyses were done with R (see above) using the packages stats , graphics , lattice , pgirmess , gplots and car . Normality and homoscedasticity were tested with the Shapiro-Wilk and Levene test, respectively, and nonparametric statistics used when these assumptions were not met. For all statistical tests, a significance threshold of α =0.05 was set. TRLC (62 d.p.i.) was compared between species using ANOVA followed by a post hoc Tukey HSD test, whereas for the er hyphae length (62 d.p.i.) a Kruskal–Wallis test followed by a post hoc Kruskal mc test (R package pgirmess ) was performed. Total aboveground biomass (as dry weight) was modelled using generalized linear models (GLMs) with Species (5 factor levels: Pl , Pm , Vc , Mt , Pa ) and Treatment (2 factor levels: NM, AM) as factors. Foliar P, C and N content as well as the number of metabolic features per sample were fitted with GLMs using Biomass as covariate and Species and Treatment as factors. Therefore, depending on the data distribution, different combinations of error structures (Gaussian, gamma) and link functions (identity, inverse, log) were used. Starting with the saturated models including all covariates, factors and their interactions, minimal adequate models were obtained by backward stepwise progression (‘model simplification’) using Akaike’s information criterion. Analysis of deviance tables with F (Gaussian) or χ 2 (gamma) statistics and terms added sequentially were constructed. Treatment contrast tables were constructed using the factor levels Pl ( Species ) and NM ( Treatment ) as reference group. Note that for treatment contrasts, estimates are given on the scale of the link function. Model fit was assessed by diagnostics of deviance residuals and inspection of predicted values. Intensities of individual metabolic features were compared between AM and NM plants within each species using two-sided Mann–Whitney U -tests, and P values corrected for multiple testing according to Benjamini and Hochberg [47] at a false discovery rate of FDR=0.05 within each species. A Venn diagram (R package gplots ) for the numbers of metabolic features in each species and the overlaps between species was constructed. Furthermore, all metabolic features were included in a PCA after autoscaling (that is, mean-centering and scaling to unit variance). Volcano plots [48] including all metabolic features of a given plant species with fold changes (mean intensity in mycorrhizal plants divided by mean intensity in control plants, presented on a log 2 scale for symmetry) were plotted in MATLAB (7.10.0.499; The MathWorks, Natick, MA, USA). To take into account that multiple testing may influence the results, all metabolic features had to pass two thresholds, namely unadjusted P values<0.05 (Mann–Whitney U -tests) as well as a fold change <0.67 (corresponding to<−0.58 on a log 2 scale) for a decrease in metabolite pool size or >1.5 (>0.58 on a log 2 scale) for an increase in metabolite pool size to be considered as modulated by AM, according to Fester et al. [6] These thresholds were set with unadjusted P values, since adjustments (which are also given) are highly conservative due to the large numbers of metabolic features (see above). For each species, a χ 2 -test was performed to test whether the number of decreased and increased features differed from a uniform distribution. A cluster heatmap including log 2 -scaled fold changes of all features being modulated by AMF according to both mentioned thresholds in at least one plant species was constructed to depict whether features were changed in the same direction in other species as well, although not significantly. Therefore, average linkage hierarchical clustering relying on the Pearson correlation distance matrices clustering both over species and metabolic features was performed with Cluster 3.0 (ref. 49 ) and heatmaps visualized with JavaTreeView [50] . Metabolic features occurring exclusively in NM or AM plants within a species, that is, features changed in a qualitative manner, were set to maximum fold changes observed for other features and included in the heatmaps. A metabolic map was constructed using KEGG reference pathways [51] complemented with information on biosynthesis of iridoids [33] , verbascoside [52] , and pinitol [53] . How to cite this article: Schweiger, R. et al. High specificity in plant leaf metabolic responses to arbuscular mycorrhiza. Nat. Commun. 5:3886 doi: 10.1038/ncomms4886 (2014).